Site-specific mapping and quantification of proteinS-sulphenylation in cells Cysteine S -sulphenylation provides redox regulation of protein functions, but the global cellular impact of this transient post-translational modification remains unexplored. We describe a chemoproteomic workflow to map and quantify over 1,000 S -sulphenylation sites on more than 700 proteins in intact cells. Quantitative analysis of human cells stimulated with hydrogen peroxide or epidermal growth factor measured hundreds of site selective redox changes. Different cysteines in the same proteins displayed dramatic differences in susceptibility to S- sulphenylation. Newly discovered S -sulphenylations provided mechanistic support for proposed cysteine redox reactions and suggested novel redox mechanisms, including S -sulphenyl-mediated redox regulation of the transcription factor HIF1A by SIRT6. S -sulphenylation is favored at solvent-exposed protein surfaces and is associated with sequence motifs that are distinct from those for other thiol modifications. S -sulphenylations affect regulators of phosphorylation, acetylation and ubiquitylation, which suggest regulatory crosstalk between redox control and signalling pathways. Protein S -sulphenylation, the reversible oxidation of protein cysteinyl thiols to suphenic acids (R-SOH), has emerged as a potential mechanism to regulate protein functions, signal transduction and effects of oxidative stress [1] . Because of its intrinsically unstable nature, protein S -sulphenylation previously has been detected indirectly by monitoring loss of reactivity with thiol-modifying reagents [2] . Recently, the use of the β-dicarbonyl compound dimedone and its analogues has enabled selective labelling and detection of protein S -sulphenylation [1] . This strategy has expanded the catalogue of proteins that apparently undergo S -sulphenylation. For example, Paulsen et al. [3] reported that the use a clickable dimedone-base probe, DYn-2, to detect S -suphenylated proteins in human cells and demonstrated that a critical active site cysteine (Cys797) on the EGF receptor is directly S -suphenylated by H 2 O 2 induced through growth factor stimulation. Using the same probe, Kulathu et al. [4] found that many ovarian tumour deubiquitinases undergo S -sulphenylation on treatment with H 2 O 2 . Leonard et al. [5] used an azide analogue of dimedone for selective labelling, capture by Staudinger ligation, and identification of S -sulphenylated proteins in cells by liquid chromatography-tandem mass spectrometry (LC-MS/MS). They identified 193 proteins as apparent targets of protein S -sulphenylation, but no specific sites of modification were reported. Major limitations of such protein-level identifications are false-positive identifications due to nonspecifically captured proteins and a lack of information about the sites and multiplicity of redox changes. Only site-specific mapping of S -suphenylated residues provides definitive confirmation. A method for global identification and quantitation of S -suphenylated residues would enable comprehensive assessment of this redox modification in cell systems. We and others have recently reported several chemoproteomic strategies for identifying protein modification sites with various clickable probes (azide or alkyne chemicals) [6] , [7] , [8] , [9] , [10] , [11] . Typically, cells or protein extracts are first labelled with the probe and the labelled proteins then are tagged with a functionalized biotin reagent containing a cleavable linker via Cu I -catalyzed azide-alkyne cycloaddition reaction (CuAAC, click chemistry). After tryptic digestion, modified peptides are enriched by biotin–streptavidin affinity and analysed by LC-MS/MS. Although it has been applied to analyse protein extracts labelled with probes in vitro, this approach has never been optimized for global, site-specific mapping and quantitation of low-abundance chemical modifications in intact cellular systems. This challenge thus presents a barrier to the study of labile redox modifications in cells. Here, we describe the use of this selective cysteine sulphenic acid labelling technique in a highly efficient chemoproteomics workflow ( Fig. 1a ) to globally map the sites of protein S -sulphenylation in cultured cells. The strategy can identify ~1,000 protein S -sulphenylation events for a single cellular condition. Moreover, we quantitatively measure hundreds of dynamic cellular S -sulphenylation changes in response to either exogenous H 2 O 2 or growth factor stimulation. Functional analysis of a novel S -sulphenylated site on SIRT6 protein reveals an unexpected role of this histone deacetylase as a potential redox sensor and transducer. Bioinformatic and structural analyses indicates that protein S -sulphenylation can impact many biological and functional categories and has distinct structural features. 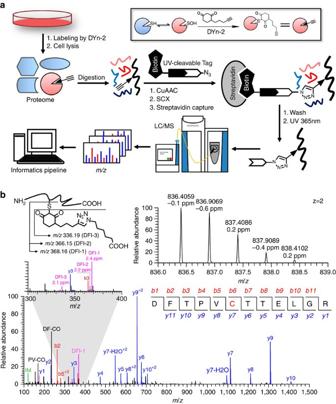Figure 1: Site-specific mapping of proteinS-sulphenylation in cells. (a) Workflow for selective labelling and analysis of proteinS-sulphenylation in living cells.S-sulphenylated cysteines in intact RKO cells were labelled with the dimedone-based probe, DYn-2. Cell proteins then were digested with trypsin and labelled peptides were conjugated with azide biotin reagent, captured with streptavidin beads, and released by photocleavage of the biotin linker. The released DYn-2-triazohexanoic acid-modified peptides were analysed by LC-MS/MS. (b) Characteristic fragmentation of modified peptides (upper, left) and a representative MS1 spectrum (upper, right) and HCD MS/MS spectrum (lower) of a DYn-2-triazohexanoic acid-modified peptide fromS-sulphenylated PRDX6. The highlighted cysteine in the peptide sequence represents theS-sulphenylated site (C47) of PRDX6. A zoom window displays the high mass accuracy of three DFI peaks. Figure 1: Site-specific mapping of protein S -sulphenylation in cells. ( a ) Workflow for selective labelling and analysis of protein S -sulphenylation in living cells. S -sulphenylated cysteines in intact RKO cells were labelled with the dimedone-based probe, DYn-2. Cell proteins then were digested with trypsin and labelled peptides were conjugated with azide biotin reagent, captured with streptavidin beads, and released by photocleavage of the biotin linker. The released DYn-2-triazohexanoic acid-modified peptides were analysed by LC-MS/MS. ( b ) Characteristic fragmentation of modified peptides (upper, left) and a representative MS1 spectrum (upper, right) and HCD MS/MS spectrum (lower) of a DYn-2-triazohexanoic acid-modified peptide from S -sulphenylated PRDX6. The highlighted cysteine in the peptide sequence represents the S -sulphenylated site (C47) of PRDX6. A zoom window displays the high mass accuracy of three DFI peaks. Full size image Site-specific mapping of protein S -sulphenylation in cells First, we optimized a method for modified peptide capture based on our previously reported chemoproteomic protocol [6] . The major challenge we faced was to improve the efficiency of click derivatization of DYn-2-labelled peptides. Given the literature precedent of poor performance under aqueous conditions of tris[(1-benzyl-1H-1,2,3-triazol-4-yl)methyl]amine (TBTA), the ligand most widely used for CuAAC acceleration [12] , we focused on improvements in the CuAAC reaction to ensure high yields in linking the alkynyl tag to azido biotinylated peptide. The new protocol has three features: (i) TBTA and the other reagents are dissolved thoroughly in the reaction solvent containing 30% acetonitrile (ACN) in mild acid, (ii) a high catalyst concentration is used and (iii) the CuAAC reaction is performed after tryptic digestion and excess biotin reagents are removed by strong cation exchange (SCX). We also optimized the procedures for washing streptavidin-captured peptides to minimize interferences from TBTA and byproducts of CuAAC reaction. We then used the optimized workflow, termed SulfenM, with a selective cysteine sulphenic acid labelling probe, DYn-2 (ref. 3 ), to site specifically map the sites of protein S -sulphenylation in RKO colon adenocarcinoma cells. We detected 1,153 distinct S -sulphenylated peptides ( Supplementary Dataset 1 ) using high-energy collisional dissociation (HCD) MS/MS [13] on a Q-Exactive MS instrument, which provides full mass range peptide fragmentation with high mass accuracy, greatly aiding precise identification. The mass errors for the precursor and fragment ions of modified peptides were within the range of 5 and 20 p.p.m., respectively ( Supplementary Fig. 1 ). In addition, we found that the DYn-2/click-derived modification produced several major diagnostic fragment ions (DFIs) at m/z 368.16, 366.15, 336.19 ( Fig. 1b ), which are generated by fragmentations analogous to those reported for cysteine conjugates [14] . We observed that all HCD spectra of DYn-2/click-modified peptides contain DFIs, which increase the confidence of S -sulphenylated peptide identifications. Furthermore, we designed a decision-tree approach for validation of peptide-spectrum matches (PSM; Supplementary Fig. 2 ), which yields 952 fully localized S -sulphenylated sites on 680 proteins ( Supplementary Dataset 2 ). We further verified several novel protein targets of S -sulphenylation, including ACTN, ACLY, CFL1 EEF1G, MAPK1, HSP90, RPL18, SIRT6, TUBB and YWAHE by a combination of affinity purification and western blotting ( Supplementary Fig. 3 ). Quantitative analysis of the S -sulphenylome in cells Next, we adapted our approach to quantify alterations in global S -sulphenylation in response to stimuli ( Fig. 2a ). In this strategy, termed SulfenQ, cells in two different conditions are labelled with light and heavy DYn-2 isotopomers, then combined and digested with trypsin. Tagged peptides are biotinylated, captured and enriched as described above. The relative change in protein S -sulphenylation between two conditions is determined by the ratio of extracted ion current peak intensities for heavy and light isotope-labelled DYn-2-tagged peptides, using the MS1 filtering function of Skyline software [15] . We first verified the accuracy of SulfenQ by mixing varying amounts of light or heavy DYn-2-labelled RKO proteomes in different ratios (L:H=1:4, 1:1, 4:1). The observed signals for labelled S -sulphenylated peptides closely matched the expected ratios ( Supplementary Fig. 4 ). 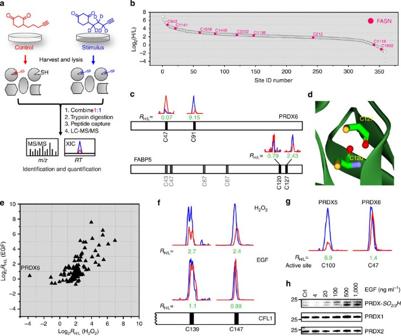Figure 2: QuantitativeS-sulphenylome analyses in cells. (a) Schematic representation of SulfenQ strategy. Intact cells treated with or without H2O2were labelled with heavy and light DYn-2, respectively, lysed and mixed at a 1:1 ratio for tryptic digestion andS-sulphenylated peptide capture. (b) The proteome-wide and site-specific changes inS-sulphenylation in intact RKO cells in response to exogenous H2O2(500 μM, 5 min), where nineS-sulphenylated cysteines on the FASN protein are shown in red, and all other cysteines by white symbols. Ratios of heavy- to light- isotope-labelled peak intensities (H2O2versus control) are displayed on a log2 scale on theyaxis. (c) Extracted ion chromatograms are shown for changes inS-sulphenylated peptides from PRDX6 (top) and FABP5 (bottom) from H2O2stimulation in RKO cells, with the profiles for light- and heavy- labelled peptides in red and blue, respectively. The site location and the experimental ratios calculated from at least four replicates are displayed below the individual chromatograms, respectively. (d) Two adjacent cysteine residues (C120 and C127, yellow colour) were mapped onto the crystal structure of FABP5 (protein databank structure 4AZM). The structure was visualized using Discovery studio. (e) Analysis ofS-sulphenylome changes induced by endogenous H2O2production on EGF stimulation and its correlation with that produced by exogenous H2O2. Log2RH/Lvalues of the intensity ofS-sulphenylated peptides identified using EGF (100 ng ml−1, 5 min) as stimulus in A431 cells are plotted against those of data from H2O2treatment, as shown inFig. 2b. Only peptides identified asS-sulphenyl sites in both datasets are included. (f) Comparison of XICs ofS-sulphenylated peptides from CFL1 on EGF and H2O2treatment. (g) XICs ofS-sulphenylated peptides from PRDX5 (2-Cys peroxiredoxin) and PRDX6 (1-Cys peroxiredoxin) on EGF stimulation in A431 cells. (h) Levels of over-oxidized peroxiredoxins in A431 cells were treated with different concentrations of EGF for 5 min. Peroxiredoxins with the same catalytic sequence (PRDX1-4) were detected by immunoblotting using anti-peroxiredoxin-SO2/3H antibody. PRDX1 and PRDX2 were also immunoblotted as protein expression controls. Full-length gels are shown inSupplementary Fig. 11. Figure 2: Quantitative S -sulphenylome analyses in cells. ( a ) Schematic representation of SulfenQ strategy. Intact cells treated with or without H 2 O 2 were labelled with heavy and light DYn-2, respectively, lysed and mixed at a 1:1 ratio for tryptic digestion and S -sulphenylated peptide capture. ( b ) The proteome-wide and site-specific changes in S -sulphenylation in intact RKO cells in response to exogenous H 2 O 2 (500 μM, 5 min), where nine S -sulphenylated cysteines on the FASN protein are shown in red, and all other cysteines by white symbols. Ratios of heavy- to light- isotope-labelled peak intensities (H 2 O 2 versus control) are displayed on a log2 scale on the y axis. ( c ) Extracted ion chromatograms are shown for changes in S -sulphenylated peptides from PRDX6 (top) and FABP5 (bottom) from H 2 O 2 stimulation in RKO cells, with the profiles for light- and heavy- labelled peptides in red and blue, respectively. The site location and the experimental ratios calculated from at least four replicates are displayed below the individual chromatograms, respectively. ( d ) Two adjacent cysteine residues (C120 and C127, yellow colour) were mapped onto the crystal structure of FABP5 (protein databank structure 4AZM). The structure was visualized using Discovery studio. ( e ) Analysis of S -sulphenylome changes induced by endogenous H 2 O 2 production on EGF stimulation and its correlation with that produced by exogenous H 2 O 2 . Log 2 R H/L values of the intensity of S -sulphenylated peptides identified using EGF (100 ng ml −1 , 5 min) as stimulus in A431 cells are plotted against those of data from H 2 O 2 treatment, as shown in Fig. 2b . Only peptides identified as S -sulphenyl sites in both datasets are included. ( f ) Comparison of XICs of S -sulphenylated peptides from CFL1 on EGF and H 2 O 2 treatment. ( g ) XICs of S -sulphenylated peptides from PRDX5 (2-Cys peroxiredoxin) and PRDX6 (1-Cys peroxiredoxin) on EGF stimulation in A431 cells. ( h ) Levels of over-oxidized peroxiredoxins in A431 cells were treated with different concentrations of EGF for 5 min. Peroxiredoxins with the same catalytic sequence (PRDX1-4) were detected by immunoblotting using anti-peroxiredoxin-SO 2/3 H antibody. PRDX1 and PRDX2 were also immunoblotted as protein expression controls. Full-length gels are shown in Supplementary Fig. 11 . Full size image We measured S -sulphenylation changes produced in RKO cells by the prototypical oxidant hydrogen peroxide (H 2 O 2 ), which also plays essential regulatory roles in multiple cellular processes [16] . We observed dramatic changes in the S -sulphenylome on H 2 O 2 treatment, with an increase of >twofold in the intensities of >89% of modified sites ( Fig. 2b , Supplementary Fig. 5 and Supplementary Dataset 3 ). We also noted that multiple S -sulphenylated sites on the same protein could sense exogenous H 2 O 2 in a markedly different manner. For example, ratios of R H/L of nine cysteines on fatty acid synthase (FASN) distributed broadly over a >60-fold range ( Fig. 2b , Supplementary Fig. 6 ). Of two cysteine residues on PRDX6 ( Fig. 2c ), C91 showed dramatic increase in S-sulphenylation after H 2 O 2 treatment ( R H/L =9.15), whereas the PRDX6 active site C47 showed opposite behaviour ( R H/L =0.07), in agreement with the well-known susceptibility of the active site of this 1-Cys peroxiredoxin to overoxidation (to Cys-SO 2 H or Cys-SO 3 H). Furthermore, changes in S -sulphenylation of two adjacent cysteine residues (C120 and C127, Fig. 2d ) on the epidermal fatty acid binding protein FABP5 were also strikingly different in response to H 2 O 2 ( Fig. 2c ). C127 was more highly S -sulphenylated after H 2 O 2 treatment ( R H/L =2.43), whereas S -sulphenylation on C120 remained almost unchanged ( R H/L =0.79). This finding might suggest that S -sulphenylation of C127, rather than C120, was responsible for a disulphide bond formation within the ligand binding cavity of FABP5, which was proposed to be crucial for its biological activity [17] . The foregoing experiments led us to further explore S -sulphenylome changes by cellular H 2 O 2 production in response to growth factor signalling. Accordingly, we investigated the EGF-dependent changes in protein S -sulphenylation in a global and site-specific manner. As expected, we observed dramatic changes in the S -sulphenylome on EGF treatment in A431 cells (100 ng ml −1 , 5 min), with an increase of >twofold in the intensities of approximately half of the detected sites ( Supplementary Fig. 7 and Supplementary Dataset 4 ), whereas the remaining sites were unchanged (0.5<R<2). In contrast, H 2 O 2 produced significant changes in over 90% of detected S -sulphenyl sites. Although global S -sulphenylation changes induced by EGF correlated well with those produced by exogenous H 2 O 2 ( Fig. 2e ), the endogenous, EGF-driven oxidative perturbation was considerably more selective and specific. For example, as shown in Fig. 2f , S -sulphenylation of two cysteines on cofilin 1 (CFL1) protein (C139 and C147) was increased by H 2 O 2 treatment (R H/L =2.7 and 2.4, respectively), whereas their S -sulphenyl forms were not changed by EGF treatment (R H/L =1.1 and 0.89, respectively). Surprisingly, S -sulphenylation of the catalytic C47 residue PRDX6 was unchanged in A431 cells treated with EGF, whereas S -sulphenylation of the catalytic site C100 on the 2-Cys peroxiredoxin PRDX5 was increased 6.9-fold, suggesting that these highly nucleophilic sites are not over-oxidized to sulphinic acid (−SO 2 H) or sulphonic acid (−SO 3 H) by endogenous oxidants ( Fig. 2g ). We also observed that 5 min treatment in A431 cells with 100 ng ml −1 EGF does not induce overoxidation on PRDX1 or PRDX2 ( Fig. 2h ). Since peroxiredoxins maintain control of protein redox homeostasis, their resistance to endogenous oxidant production may confer relative stability of the cellular S -sulphenylome in response to physiologic stimuli. Functional analysis of S -sulphenylation on SIRT6 Among the most highly and consistently S -sulphenylated proteins was SIRT6, a member of a conserved family of NAD + -dependent deacetylases with important functions in cellular metabolism, stress resistance and cancer [18] , [19] , [20] , [21] ( Fig. 3a,b ). SIRT6 functions as a corepressor of HIF1A, thereby regulating glucose homeostasis, but the molecular basis of their interaction is still unclear [22] . Among the five cysteine residues on SIRT6, Cys18 was exclusively and highly S -sulphenylated ( Supplementary Dataset 2 ). We thus hypothesized that SIRT6 binds HIF1A in a redox-dependent manner. To test this hypothesis, we incubated human recombinant SIRT6 with HIF1A protein fragment (530–826), which contains three cysteines, with or without H 2 O 2 . We then analysed the complexes by electrophoresis and western blotting. Without H 2 O 2 treatment, SIRT6 migrated as a single band corresponding to its monomeric form ( Fig. 3c ). On H 2 O 2 treatment in the presence of HIF1A, SIRT6 migrated at higher apparent molecular weights, particularly in non-reducing gels ( Fig. 3c ). HIF1A migration displayed similar H 2 O 2 -dependent migration in the presence of SIRT6 ( Fig. 3c ). These results suggested that an intermolecular disulphide bond was formed between SIRT6 and HIF1A. Moreover, treatment with dimedone, a cysteine sulphenic acid labelling reagent, abolished these mobility shifts ( Fig. 3d ), suggesting that this oxidative aggregation is initiated by an S -sulphenylation event. We further analysed the mixture by LC-MS/MS to identify the specific S -sulphenylation event on SIRT6 responsible for intermolecular disulphide bond formation between SIRT6 and HIF1A. An ion with a mass matching the theoretical mass of disulphide-linked peptides 18–24 of SIRT6 and 799–810 of HIF1A was detected ( Fig. 3e , inset). MS/MS fragmentation of this peptide ion further confirmed the expected SIRT6 and HIF1A sequences ( Fig. 3e ). Taken together, these data establish that the SIRT6–HIF1A disulphide linkage is formed between Cys18 (SIRT6) and Cys800 (HIF1A; Fig. 3f ) and is mediated by cysteine S -sulphenylation. This result suggests that SIRT6 may exert redox control of HIF1A transcriptional activity through reversible formation of disulphide-linked SIRT6–HIF1A complex. 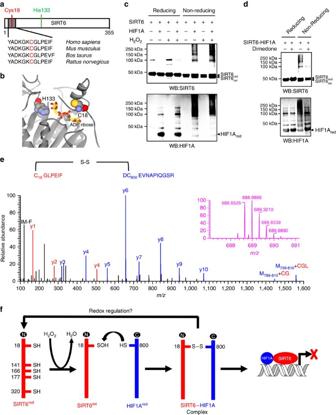Figure 3: Functional analysis ofS-sulphenylation on SIRT6. (a) TheS-sulphenylation site Cys18 near the amino terminus of SIRT6 is evolutionarily conserved. (b) TheS-sulphenylation site and the active site of SIRT6 were mapped onto the crystal structure of SIRT6 (PDB#: 3PKI) and visualized with Discovery Studio. (c) Human recombinant SIRT6 forms reducible, covalent complexes with HIF1A on treatment with H2O2. Mixtures of the proteins were incubated with or without 0.5 mM H2O2at 37 °C. After 4 h incubation, the reaction mixtures were analysed by reducing or non-reducing SDS-polyacrylamide gel electrophoresis gels and SIRT6 (upper) or HIF1A (lower) complexes were detected by immunoblotting. (d) Dimedone inhibits intermolecular disulphide formation between SIRT6 and HIF1A. H2O2treated SIRT6–HIF1A mixtures were incubated in the presence or absence of 10 mM dimedone at 37 °C for 4 h and SIRT6 (upper) or HIF1A (lower) complexes were detected by immunoblotting. (e) Identification of the cysteines involved in the intermolecular disulphide formation between SIRT6 and HIF1A. Human recombinant SIRT6 and HIF1A fragment (530–826) were incubated with 0.5 mM H2O2at 37 °C. After 4 h incubation, the reaction mixture was digested with trypsin and then with AspN and analysed by LC-MS/MS. The MS/MS fragment ions of SIRT6 peptide (18–24) and HIF1A peptide (799–810) are depicted in red and blue, respectively. Inset shows the high-resolution MS spectrum of the disulphide-linked peptide from the SIRT6–HIF1A complex. (f) Hypothetical model for the redox-based gene regulatory interaction between SIRT6 and HIF1A. Figure 3: Functional analysis of S -sulphenylation on SIRT6. ( a ) The S -sulphenylation site Cys18 near the amino terminus of SIRT6 is evolutionarily conserved. ( b ) The S -sulphenylation site and the active site of SIRT6 were mapped onto the crystal structure of SIRT6 (PDB#: 3PKI) and visualized with Discovery Studio. ( c ) Human recombinant SIRT6 forms reducible, covalent complexes with HIF1A on treatment with H 2 O 2 . Mixtures of the proteins were incubated with or without 0.5 mM H 2 O 2 at 37 °C. After 4 h incubation, the reaction mixtures were analysed by reducing or non-reducing SDS-polyacrylamide gel electrophoresis gels and SIRT6 (upper) or HIF1A (lower) complexes were detected by immunoblotting. ( d ) Dimedone inhibits intermolecular disulphide formation between SIRT6 and HIF1A. H 2 O 2 treated SIRT6–HIF1A mixtures were incubated in the presence or absence of 10 mM dimedone at 37 °C for 4 h and SIRT6 (upper) or HIF1A (lower) complexes were detected by immunoblotting. ( e ) Identification of the cysteines involved in the intermolecular disulphide formation between SIRT6 and HIF1A. Human recombinant SIRT6 and HIF1A fragment (530–826) were incubated with 0.5 mM H 2 O 2 at 37 °C. After 4 h incubation, the reaction mixture was digested with trypsin and then with AspN and analysed by LC-MS/MS. The MS/MS fragment ions of SIRT6 peptide (18–24) and HIF1A peptide (799–810) are depicted in red and blue, respectively. Inset shows the high-resolution MS spectrum of the disulphide-linked peptide from the SIRT6–HIF1A complex. ( f ) Hypothetical model for the redox-based gene regulatory interaction between SIRT6 and HIF1A. Full size image Bioinformatics analysis of the S -sulphenylome To better understand the systems impact of protein S -sulphenylation, we used DAVID software [23] to perform several bioinformatics enrichment analyses of the S -sulphenylome detected in RKO cells. S -sulphenylated proteins are widely distributed across all major cellular compartments ( Fig. 4a ) and represent diverse cellular processes and pathways ( Fig. 4b ). A large number of S -sulphenylated proteins are present in the nucleus ( Fig. 4a ) and represent most major nuclear processes, including RNA processing, translation, transportation and cell cycle ( Fig. 4b ). We did not detect S -sulphenylation of redox-sensitive transcription factors, which are believed to function as the important determinants of proper redox state in the nucleus [24] . This may reflect the low abundance of many transcription factors, such that detection of their S -sulphenyl peptides is suppressed by the presence of more abundant S -sulphenyl peptides. In addition, extensively S -sulphenylated nuclear proteins, such as EEF1A1, NTMT1 and SIRT6, may function as H 2 O 2 sensors that then interact with transcription factors, thus enabling redox regulation through thiol-disulphide exchange, rather than direct oxidation by H 2 O 2 (ref. 25 ). 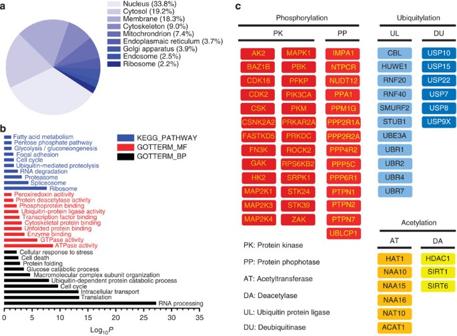Figure 4: GO classification of theS-sulphenylome. (a) Cellular compartment terms associated with sulphenylated proteins. (b) GO annotations enriched inS-sulphenylome. (c) Occurrence ofS-sulphenylation sites on proteins associated with post-translational regulation of cell signaling. Figure 4: GO classification of the S -sulphenylome. ( a ) Cellular compartment terms associated with sulphenylated proteins. ( b ) GO annotations enriched in S -sulphenylome. ( c ) Occurrence of S -sulphenylation sites on proteins associated with post-translational regulation of cell signaling. Full size image Gene ontology (GO) classification and KEGG pathway analysis revealed enrichment of S -sulphenylated proteins involved in protein deubiquitination (GO_BP, P =9.1 × 10 −9 ; GO_MF, P =2.9 × 10 −3 ; KEGG, P =1.8 × 10 −2 ). Together with recent studies that show deubiquitinases can be targeted and regulated by S -sulphenylation [4] , [26] , these findings strongly suggest that protein ubiquitination may be influenced by redox regulation. We also noted that S -sulphenylated proteins were enriched in several biological processes and pathways involving cell metabolism, including glucose catabolic processes (GO_BP, P =3.2 × 10 −4 ), glycolysis (KEGG, P =4.5 × 10 −2 ), pentose phosphate pathway (KEGG, P =4.6 × 10 −2 ) and fatty acid metabolism (KEGG, P =6.6 × 10 −2 ). In particular, pyruvate kinase M2 (PKM2), a glycolytic enzyme, was S -sulphenylated on three cysteine residues (C49, C358 and C423/424) under basal conditions. One of these (C358) was found to be critical for metabolic reprogramming regulated by PKM2 via reversible oxidation during cancer development [27] . In another example, S -sulphenylation of C212 on FASN may drive intramolecular disulfide formation in the β-ketoacyl synthase domain, thereby blocking the active site (C161) for fatty acid synthesis ( Supplementary Fig. 6 ) [28] . Structure profiling of S -sulphenylated cysteine residues We identified a total of 1,105 S -sulphenylated sites on 778 proteins in RKO cells, the majority of which (92%) had only one or two S -sulphenylated residues ( Fig. 5a ). A few proteins (1.3%) were extensively oxidized (number of sites ≥5), including FASN and MKI67, both with 9 S -sulphenyl sites. We explored structural properties of the modified cysteine residues with several computational tools and available crystal structures. First, we performed a prediction analysis of the relative residue surface accessibility (RSA) for all cysteine residues (modified and unmodified) within the S -sulphenylome using NetSurfP [29] . As expected, >60% of the S -sulphenylated cysteine residues were solvent-exposed (with a relative RSA of greater than 25%), which was dramatically higher than that (<30%) for all unmodified cysteine residues within the same proteins. We also compared the probability distribution for relative RSA for S -sulphenylated cysteines with that for unmodified cysteine residues ( Fig. 5b ) and by plotting the percentile rankings against each other ( Fig. 5c ). Both analyses demonstrated that S -sulphenylated cysteine residues showed a marked tendency to reside on surface-accessible areas compared with unmodified cysteine residues, which suggests that solvent accessibility is one of the major determinants for the redox reactivity of cysteines. 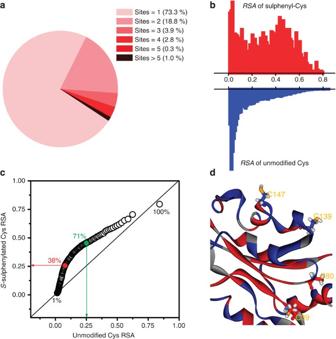Figure 5: Impact of cysteine surface accessibility onS-sulphenylation. (a) Distribution of the number ofS-sulphenylated cysteine residues per protein. (b) Distributions of the relative RSA forS-sulphenylated cysteine versus unmodified cysteine residues. (c) Q–Q plot of the relative RSA forS-sulphenylated cysteine versus unmodified cysteine residues. The relative RSA values ofS-sulphenylated and unmodified cysteine residues were predicted with NetSurfP, percentiled and sorted from 1 to 100% with a 1% interval, respectively. The RSA values at the 38th percentile were 0.25 (S-sulphenyl) versus 0.08 (unmodified) and 0.45 (S-sulphenyl) versus 0.25 (unmodified) at the 71st percentile, thus indicating thatS-sulphenylated cysteine residues are favoured at exposed protein surfaces. (d) Crystal structure of CFL1 (protein databank structure 1Q8G) with the twoS-sulphenylated cysteines (C139 and C147) mapped onto the solvent-accessible surface (Blue) and the unmodified cysteines buried (Red). Figure 5: Impact of cysteine surface accessibility on S -sulphenylation. ( a ) Distribution of the number of S -sulphenylated cysteine residues per protein. ( b ) Distributions of the relative RSA for S -sulphenylated cysteine versus unmodified cysteine residues. ( c ) Q–Q plot of the relative RSA for S -sulphenylated cysteine versus unmodified cysteine residues. The relative RSA values of S -sulphenylated and unmodified cysteine residues were predicted with NetSurfP, percentiled and sorted from 1 to 100% with a 1% interval, respectively. The RSA values at the 38th percentile were 0.25 ( S -sulphenyl) versus 0.08 (unmodified) and 0.45 ( S -sulphenyl) versus 0.25 (unmodified) at the 71st percentile, thus indicating that S -sulphenylated cysteine residues are favoured at exposed protein surfaces. ( d ) Crystal structure of CFL1 (protein databank structure 1Q8G) with the two S -sulphenylated cysteines (C139 and C147) mapped onto the solvent-accessible surface (Blue) and the unmodified cysteines buried (Red). Full size image To further confirm this finding, we mapped identified S -sulphenylated sites onto several proteins with available crystal structures and calculated solvent accessibilities with a default probe radius of 1.4 Å. For example, among four cysteines on human CFL1, only two highly solvent-accessible residues, C139 and C147 ( Fig. 5d ), were found to be targeted by S -sulphenylation under both basal and stimulated conditions. In another example, the highly exposed catalytic cysteine residue, C152, of GAPDH also was highly S -sulphenylated, even under basal oxidation conditions ( Supplementary Fig. 8 ). However, S -sulphenylation of C247, one of the buried cysteine residues within GAPDH, was still detectable, although much less abundant ( Supplementary Fig. 8 ), in accordance with an earlier study of thiol reactivity in GAPDH [30] . We should note that the detection of S -sulphenylation requires that our probe be able to react with the oxidized residue and that steric features may hinder labelling of some S -sulphenylated cysteines. Accordingly, our conclusion regarding the potential surface-localization tendency of S -sulphenylation may be biased somewhat by an unavoidable limitation of chemical labelling strategy. To further explore structural features that may define protein S -sulphenylation, we examined flanking sequences of S -sulphenylated cysteine residues with the pLogo algorithm for the presence of linear motifs and we further compared these with motifs associated with other cysteine modifications, such as S -nitrosylation [31] and electrophile-based alkylation [7] . Strikingly, S -sulphenylated cysteines resided within consensus motifs with features distinct from those for S -nitrosylated and electrophile-sensitive cysteines. Specifically, Glu was significantly overrepresented at the −4, −3, +1, +3, +4 and +5 position of S -sulphenylation sites, whereas Lys was significantly overrepresented at the −6, −5, −2 and +6 position ( P <0.05, Fig. 6 ). Notably, Glu and Lys have complementary physiochemical properties (Glu is negatively charged and acts as a hydrogen acceptor, whereas Lys is a positively charged and acts as a hydrogen donor). Protonated Glu may be capable of reducing the pKa of an adjacent thiol via hydrogen bond formation [32] . Glu was highly represented in the +3 and +4 positions of S -sulphenylated sites ( Fig. 6 ) and is also highly conserved at the +3 position adjacent to the catalytic cysteines of all the 2-Cys peroxiredoxins, the best-known targets of H 2 O 2 . We also found that Cys is largely absent in consensus flanking sequences of all the aforementioned cysteine modifications ( Fig. 6 ). Indeed, the absence of adjacent cysteines is considered to be the major stabilizing factor for cysteine sulphenic acid [33] . 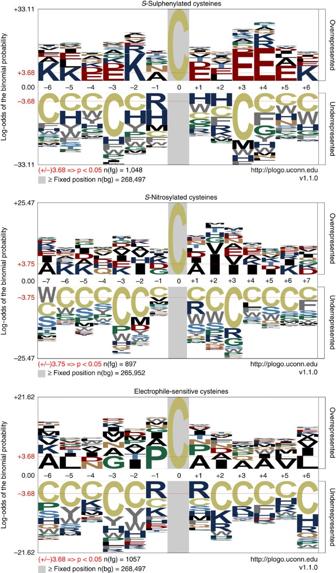Figure 6: Sequence motif analysis of proteinS-sulphenylation. Comparison of calculated sequence motif forS-sulphenylated (1,048, human),S-nitrosylated (897, mouse) and electrophile-alkylated cysteines (1,057, human). Images were generated with pLogo and scaled to the height of the largest column within the sequence visualization. The red horizontal lines on the pLogo plots denoteP=0.05 thresholds. Figure 6: Sequence motif analysis of protein S -sulphenylation. Comparison of calculated sequence motif for S -sulphenylated (1,048, human), S -nitrosylated (897, mouse) and electrophile-alkylated cysteines (1,057, human). Images were generated with pLogo and scaled to the height of the largest column within the sequence visualization. The red horizontal lines on the pLogo plots denote P =0.05 thresholds. Full size image Here, we describe a highly efficient chemoproteomics platform, which we applied to quantitative S -sulphenylome analysis in intact cells. In total, we identified over 1,000 S -sulphenylation sites on more than 700 proteins ( Supplementary Datasets 2–4 ), which demonstrates the potential of this platform for further systematic study of biologically relevant S -sulphenylation events. To our knowledge, the current dataset encompasses most known S -sulphenylated sites and proteins in mammalian cells and expands by two orders of magnitude the number of such sites previously listed in Uniprot. The use of DFI in MS/MS spectra and our decision-tree validation procedure ensures that these site assignments are of high reliability. Although the DYn-2 probe labelled diverse sequences, there are limitations to the labelling approach. Some S -sulphenylated cysteines may be inaccessible to the DYn-2 probe for steric reasons or because rapid formation of intramolecular bonds, such as disulphide (for example, 2-Cys PRDXs) and sulphnylamide [34] (for example, PTP1B) blocks reaction of DYn-2 with transient sulphenic acids in these proteins. A particularly important aspect of our approach is that we achieve site-specific mapping of large numbers of modifications in intact cells. Most previous studies of cysteinyl modifications were done with cell lysates treated with much higher concentrations of thiol-modifying agents [35] , [36] , [37] . A key assumption in S -sulphenylation analysis by DYn-2 labelling is that the 2 h probe labelling treatment itself does not induce oxidative stress sufficient to perturb cellular redox state. This has been established by previous experiments, which demonstrated that DYn-2 does not alter cell viability, glutathione redox balance or generate reactive oxygen species under the same labelling conditions described here [3] . Moreover, DYn-2 labelling does not result in overoxidation of peroxiredoxins ( Supplementary Fig. 9 ). Some recently published reports revealed that biological functions of a few proteins, such as CFL1 (ref. 38 ), PKM2 (ref. 27 ) and superoxide dismutase 1 (ref. 39 ) can be regulated by redox reactions, which were interpreted as reversible cysteine oxidations. Our identification of specific S -sulphenylation sites on these proteins provides further support for this hypothesis. For instance, of four cysteine residues on human CFL1, only C139 and C147 were found to be sensitive to oxidative stress and responsible for CFL1-induced mitochondrial damage [38] . We detected S -sulphenylation of only these two cysteines on CFL1 protein and also confirmed these by an orthogonal approach ( Supplementary Fig. 3d,e ). In addition, functional analysis of a novel S -sulphenylated site at SIRT6 C18, near the amino terminus of the protein, revealed a redox-dependent mechanism for interaction between SIRT6 and the transcriptional factor HIF1A ( Fig. 3 ). We found S -sulphenylated sites on the functional domains of protein kinases, phosphatases, acetyltransferases, deacetylases and deubiquitinases ( Fig. 4c ), suggesting the possibility of regulatory crosstalk between S -sulphenylation and other major post-translational modification events. Indeed, other recent studies suggest the potential regulatory impact of reversible cysteine oxidation on protein phosphorylation [3] , [40] , acetylation [41] and ubiquitylation [4] , [26] , [42] . In addition, GO annotations show that these S -sulphenylated proteins are present in all major cellular compartments and are involved in various biological processes such as cell signalling, response to stress, cell cycle and cell death ( Fig. 4 ). Structural analysis revealed consensus motifs for S -sulphenylation, such as CxxE, CxxxE and KxC, and that S -sulphenylation is favoured on protein surfaces ( Figs 5 and 6 ). In addition to p K a, other structural features influencing the local stereoelectronic environment of cysteine residues may direct S-sulphenylation site specificity in vivo . The application of quantitative S -sulphenylome analysis enabled us to quantify exogenous oxidant or growth factor induced redox events in eukaryotic cells in a global and unbiased manner. The strategy we describe here should enable more comprehensive assessment of dynamic S -sulphenylation in different contexts, such as redox perturbations associated with cell signalling, metabolism, inflammation and disease processes. Moreover, adaptation of SulfenQ could enable absolute measurement of protein S -sulphenylation stoichiometry. More broadly, application of our optimized peptide capture method with other clickable chemical probes should dramatically improve site-specific characterization of other proteomic characteristics and targets. Our analysis platform should thus find broad applications in both chemical biology and drug discovery [43] . Reagents Azido-tagged biotin with or without a photocleavable linker (biotin–ultraviolet (UV)–azide and biotin–azide) were provided by Professor Ned A. Porter [6] ( Supplementary Fig. 10 ). The synthesis of these reagents is described in the Supplementary Material of ref. 6 . DYn-2 was purchased from Cayman Chemicals. DYn-2-d6 was synthesized as described in the Supplementary Methods . SCX spin columns were purchased from Nest group. Streptavidin sepharose was purchased from GE Healthcare Life Sciences. HPLC-grade water, ACN and methanol were purchased from J.T.Baker. Other chemicals and reagents were obtained from Sigma unless otherwise indicated. Antibodies against ACLY (ab40793, diluted at 1:5,000), ACTN (ab6276, diluted at 1:5,000), CFL1 (ab42824, diluted at 1:1,000), EEF1G (ab72368, diluted at 1:5,000), MAPK1/ERK2 (ab124362, diluted at 1:1,000), RPL18 (ab166711, diluted at 1:1,000), SIRT6 (ab88494, diluted at 1:2,500), TUBB (ab7792, diluted at 1:5,000), PRDX-SO 2/3 H (ab16830, diluted at 1:2,000), PRDX1 (ab15571, diluted at 1:2,000) and PRDX2 (ab15572, diluted at 1:2,000) were purchased from Abcam. Antibodies against HSP90 (CS#4874S, diluted at 1:1,000) and YWAHE/14-3-3ε (CS#9635S, diluted at 1:1,000) were purchased from Cell Signalling Technology. Cell culture and in situ labelling experiment Human RKO and A431 cells (ATCC) were maintained at 37 °C in a 5% CO 2 , humidified atmosphere and were cultured in McCoy medium (Invitrogen) and DMEM medium (Invitrogen), respectively, containing 10% FBS (Invitrogen). For qualitative S -sulphenylome analysis, cells were grown until 70–80% confluent, rinsed with PBS quickly and labelled according to a modification of a recently published protocol [44] . In brief, cells were lifted with 0.25% trypsin-EDTA (Invitrogen), collected by centrifugation at 1,500 g for 3 min, washed and resuspended in serum-free McCoy medium at a density of ~5 × 10 6 cells ml −1 . Intact cells in suspension were incubated with 5 mM sulphenic acid labelling reagent (DYn-2 in DMSO, 2% v/v) at 37 °C with rotation. After 2 h incubation, cells were collected and washed with cold PBS three times. For quantitative S -sulphenylome analysis of both RKO and A431 cells, the cells were cultured as above, rinsed with PBS quickly and placed overnight in medium without serum. After serum deprivation, RKO cells were treated with the 500 μM H 2 O 2 or vehicle for 5 min. A431 cells were treated with 100 ng ml −1 EGF or vehicle for 5 min. Treatments were stopped by removing the medium. Cells treated with and without stimulus then were labelled with DYn-2- d 6 and DYn-2, respectively For RKO cells, labelling was for 2 h; for A431 cells, labelling was for 1 h. The resulting cells were routinely examined using a TC-10 automatic cell counter (Bio-Rad) and uniformly showed greater than 95% viability after either stimuli treatment and/or probe labelling. No evidence of oxidative stress in the tested cell lines was observed during the in situ chemical labelling, in accord with our recently published studies [3] , [5] , [45] , [46] . Sample preparation Cell pellets were lysed on ice in HEPES lysis buffer (50 mM HEPES, 150 mM NaCl, 1% Igepal, pH 7.5) containing 8 mM dithiothreitol (Research Products International). The lysate was further incubated at 75 °C for 15 min to reduce the reversibly oxidized cysteines. Reduced cysteines then were alkylated with 32 mM iodoacetamide for 30 min in the dark. Protein concentrations of lysate samples were determined with the BCA assay (Pierce Thermo Fisher). For a typical qualitative S -sulphenylome analysis, ~30 mg protein was used. For a quantitative S -sulphenylome analysis, 7.5 mg light- or heavy DYn-2-labelled protein samples were combined. Protein precipitation was performed with a methanol-chloroform system (aqueous phase/methanol/chloroform, 4:4:1 (v/v/v)) [47] . Proteins were collected at the aqueous/organic phase interface as a solid disk after centrifugation at 1,400 g for 20 min at 4 °C. Liquid layers were discarded and the protein was washed twice in methanol/chloroform (1:1, v/v), followed by centrifugation at 16,000 g for 10 min at 4 °C to repellet the protein. The protein pellets were evaporated to dryness under vacuum and resuspended with 50 mM ammonium bicarbonate containing 0.2 M urea at a protein concentration of 2 mg ml −1 . Resuspended proteins were first digested with sequencing grade trypsin (Promega) at a 1:50 (enzyme/substrate) ratio overnight at 37 °C. A secondary digestion was performed by adding additional trypsin to a 1:100 (enzyme/substrate) ratio, followed by incubation at 37 °C for additional 4 h. The tryptic digests were desalted with HLB extraction cartridges (Waters). The desalted samples were then evaporated to dryness under vacuum. Click chemistry, capture and enrichment Desalted tryptic digests were reconstituted in a solution containing 30% ACN, 0.8 mM biotin–UV–azide, 8 mM sodium ascorbate, 1 mM TBTA and 8 mM CuSO 4 , pH 6. The pH of the reaction mixture was adjusted using pH-indicator strips and the mixture was incubated for 2 h at room temperature within the dark rotation. The excess biotin reagents were removed by SCX chromatography, as previously reported [48] . In brief, the sample was diluted into SCX loading buffer (5 mM KH 2 PO 4 , 25% ACN, pH 3.0), passed through the SCX spin columns and washed with several column volumes of loading buffer. The retained peptides were eluted with a series of high-salt buffers containing 100, 200 and 400 mM NaCl. Eluent was diluted 10 × with 50 mM sodium acetate buffer (NaAc, pH 4.5) and then allowed to interact with pre-washed streptavidin sepharose for 2 h at room temperature. Streptavidin sepharose then was washed with 50 mM NaAc, 50 mM NaAc containing 2 M NaCl and water twice each with votexing and/or rotation to remove non-specific binding peptides and resuspended in 25 mM ammonium bicarbonate. The suspension of streptavidin sepharose was transferred to several glass tubes (VWR), irradiated with 365 nm UV light (Entela, Upland, CA) for 2 h at room temperature with stirring. The supernatant was collected, evaporated to dryness under vacuum and stored at −20 °C until analysis. LC-MS/MS LC-MS/MS analyses were performed on a Q-Exactive hybrid quadrupole-Orbitrap mass spectrometer (Thermo Fisher Scientific) operated with an Easy-nLC1000 system (Thermo Fisher Scientific). Samples were reconstituted in 0.1% formic acid and pressure-loaded onto a 360 μm outer diameter × 75 μm inner diameter microcapillary precolumn packed with Jupiter C18 (5 μm, 300 Å, Phenomenex) and then washed with 0.1% acetic acid. The precolumn was connected to a 360 μm outer diameter × 50 μm inner diameter microcapillary analytical column packed with the ReproSil-Pur C18-AQ (3 μm, 120 Å, Dr Maisch) and equipped with an integrated electrospray emitter tip. The spray voltage was set to 1.5 kV and the heated capillary temperature to 250 °C. For qualitative analysis, two different LC gradient conditions were used. Gradient A consisted of 0–15 min, 2% B; 35 min, 15% B; 40 min, 20% B; 50 min, 30% B; 55 min, 35% B; 59–65 min, 90% B; 80–85 min, 2% B (A=water, 0.1% formic acid; B=ACN/0.1% formic acid) at a flow rate of 300 nl min −1 . Gradient B consisted of 0–10 min, 5% B; 100 min, 35% B; 120–130 min, 90% B; 140–150 min, 5% B at a flow rate of 300 nl min −1 . For quantitative analysis, gradient A was used to achieve better peak shapes. HCD MS/MS spectra were recorded in the data-dependent mode using a Top 12 method for qualitative analysis and Top 20 method for quantitative analysis, respectively. MS1 spectra were measured with a resolution of 70,000, an AGC target of 3e6 and a mass range from m/z 300 to 1,800. HCD MS/MS spectra were acquired with a resolution of 17,500, an AGC target of 2e5 and normalized collision energy of 28. Peptide m/z that triggered MS/MS scans were dynamically excluded from further MS/MS scans for 20 s. The HCD MS/MS spectra for all identified peptides are provided as Supplementary Dataset 5 and all the raw data files are available for download at both the University of California at San Diego MassIVE portal ( ftp://MSV000078777@massive.ucsd.edu/) and the National Cancer Institute Clinical Proteomic Tumour Analysis Consortium Data Portal ( https://cptac-data-portal.georgetown.edu/cptacPublic/ ). Peptide identification and site localization Raw data files were analysed by using TagRecon algorithm [49] (Version 1.4.47) against a decoy protein database consisting of forward and reversed human RefSeq database (Version 20130621). Precursor ion mass tolerance was 0.01 Da, and fragmentation tolerance was 0.1 Da for the database search. The maximum number of modifications allowed per peptide was three, as was the maximum number of missed cleavages allowed. Methionine oxidation (15.9949 Da) and cysteine modifications either by iodoacetamide (carbamidomethyl, 57.0214 Da) or by S -sulphenylcysteine tagged with DYn-2-triazohexanoic acid group (DTH, Fig. 1b , 333.1689 Da) were searched as dynamic modifications. For quantitative S -sulphenylome analysis, the heavy DTH modification on cysteine (DTH- d 6, 339.2065) was also included as dynamic modification during database searching. The maximum Q value of PSMs was adjusted to achieve either a peptide or a protein false discovery rate no greater than 5% using IDPicker software (Version 3.0.529) [50] . Because identifications based on one peptide per protein were permitted, a streamlined manual validation approach was used to establish peptide identification and site localization ( Supplementary Fig. 2 ). First, the modified peptides whose matched spectra did not contain the major three DFIs ( m/z 368.16, 366.15, and 336.19) were excluded from further consideration. MS/MS spectra of identified S -sulphenylated peptides then were annotated automatically with the SeeMS tool embedded in IDPicker software. The mass errors of the annotated peaks were required to be less than 20 p.p.m. All the automatically annotated spectra were manually evaluated according a previously published protocol for verification of automated peptide identification [51] . For identified peptides containing more than one cysteine residue, at least three DTH modification-specific fragment ions were required for unambiguous site localization. PSMs with ambiguously localized sites identified with proper peak annotation also were retained in the final dataset. Quantitative analysis For quantitative S -sulphenylome analysis, database search results were processed using Skyline software [52] according to the tutorial for MS1 full-scan filtering ( https://skyline.gs.washington.edu/labkey/wiki/home/software/Skyline/page.view?name=tutorial_ms1_filtering ). In brief, Skyline spectral libraries were generated from database searches (as described above) of the raw data files. A subset FASTA database containing all the identifications (with and/or without modification) exported from the IDPicker files then was imported into Skyline. The peptide list was further refined in Skyline by removing all unmodified peptides, as well as modified peptides with incorrect annotations. Raw files then were directly imported into Skyline in their native file format [53] . Because MS/MS spectra were obtained in data-dependent acquisition mode, peptides were not always identified by a PSM in every replicate or run. In cases where a probe-modified peptide was identified in one run, but not in another, several criteria were applied to identify the corresponding peak in the run without the peptide identification. First, the retention time of the PSM-identified peptide (indicated by ID, Supplementary Figs 4 and 5 ) was used to position a retention time window (± 3 min) across the run lacking the same peptide identification. Second, the resolution for extracting the MS1 filtering chromatogram of the target precursor ions with both light and heavy labelled peptides was set to 70,000 at 400 Th. The use of a deuterated probe could further complicate the analysis, since there is a slight difference in the elution times of light- and deuterated (heavy, d 6)- tagged peptide pairs, with the deuterated isotopomer eluting 1-2 s before the light analogue. After data import, therefore, graphical displays of chromatographic traces for the top three isotopic peaks were manually inspected for proper peak picking of MS1 filtered peptides; those with isotopic dot product scores lower than 0.8 were rejected to ensure that the correct peak pairs were identified. In addition, several criteria were used to ensure the high accuracy of quantification: (1) signal to noise (S/N) of all the detected peptides was required to be higher than five; (2) baseline separation was required between the isotopic peaks of a quantifiable peptide and unknown isobaric interference; (3) manual integration was applied if necessary. Only the most abundant isotope for each peptide was used for quantitation. Following data extraction, the ratios of peptide areas of heavy DTH adducts to their light isotopomers ( R H:L ) were calculated automatically. Quantitation results were obtained from three biological replicates with two LC-MS/MS runs for each. All details for peptide quantitation using Skyline MS1 filtering are provided in Supplementary Datasets 3,4 . Bioinformatics Relative RSA information was obtained with the prediction algorithm NetSurfP [29] (Version 1.1). AQ-Q plot was used to determine if there was enrichment for exposed or buried cysteines for S -sulphenylated versus unmodified cysteines. The consensus sequence motifs of S -sulphenylated cysteines were visualized by pLogo [54] , a linear sequence prediction algorithm based on their statistical significance ( P <0.05). The crystal structures of FABP5, CFL1, GAPDH and FASN were visualized by Discovery Studio (Version 2.5, Accelrys) and the relative RSA values for cysteine residues were calculated with a default probe radius of 1.4 Å. GO and KEGG pathway enrichment ( P <0.05) analyses were performed by using the functional annotation tool DAVID [23] . Affinity purification and western blotting RKO cells were cultured, treated with or without H 2 O 2 and labelled with DYn-2 as described above. Cells were lysed in HEPES lysis buffer in the presence of 200 U ml −1 catalase (Sigma). Cell lysate (2 mg ml −1 , 1 ml) was incubated with 100 μM azido-tagged biotin with a photocleavable linker, 1 mM sodium ascorbate, 100 μM TBTA and 1 mM CuSO 4 for 2 h in the dark at room temperature with rotation. The proteins were precipitated with chloroform/methanol system as described above. The resulting protein precipitate then was resolubilized and subjected to streptavidin pull-down. After 1.5 h incubation at room temperature, beads were washed with 1% SDS (2 × ), 4 M urea (2 × ), 1 M NaCl (1 × ) and H 2 O (2 × ). Beads were then resuspended in 25 mM ammonium bicarbonate buffer and subjected to UV photorelease as described above. The collected proteins were resolved on SDS-polyacrylamide gel electrophoresis gels and immunoblotted with antibodies as indicated. Detection was performed with the Odyssey Infrared Imaging System (Li-Cor). Alternatively, cell lysates (1 mg protein) were incubated with 2 μg antibodies overnight at 4 °C. The immune complex was then treated with 20 μl protein A/G plus agarose (Pierce) and incubated for 1 h at 4 °C. The mixture was washed three times with IP lysis/wash buffer (Pierce) and PBS once. To analyse immunoprecipitated proteins, the beads were treated with 30 μl click chemistry mix (100 μM Azido-tagged biotin without photocleavable linker, 1 mM sodium ascorbate, 100 μM TBTA, 1 mM CuSO 4 in PBS). Reactions were quenched by boiling with 15 μl LDS sample buffer (Life Technologies) for 10 min. The collected proteins were analysed as above except that the DYn-2-labelled protein was detected by fluorescent conjugated streptavidin (Life Technologies) and immunoblotting as described above. How to cite this article : Yang, J. et al. Site-specific mapping and quantification of protein S -sulphenylation in cells. Nat. Commun . 5:4776 doi: 10.1038/ncomms5776 (2014).